Dissolution and ionization of sodium superoxide in sodium–oxygen batteries With the demand for high-energy-storage devices, the rechargeable metal–oxygen battery has attracted attention recently. Sodium–oxygen batteries have been regarded as the most promising candidates because of their lower-charge overpotential compared with that of lithium–oxygen system. However, conflicting observations with different discharge products have inhibited the understanding of precise reactions in the battery. Here we demonstrate that the competition between the electrochemical and chemical reactions in sodium–oxygen batteries leads to the dissolution and ionization of sodium superoxide, liberating superoxide anion and triggering the formation of sodium peroxide dihydrate (Na 2 O 2 ·2H 2 O). On the formation of Na 2 O 2 ·2H 2 O, the charge overpotential of sodium–oxygen cells significantly increases. This verification addresses the origin of conflicting discharge products and overpotentials observed in sodium–oxygen systems. Our proposed model provides guidelines to help direct the reactions in sodium–oxygen batteries to achieve high efficiency and rechargeability. To address the increasing use of renewable energy and launch of electric vehicles, the need for rechargeable batteries with high-energy densities has been growing more rapidly than ever before [1] , [2] . Among the available battery chemistries, metal–oxygen systems offer the highest energy density with the largest theoretical capacities. Unlike conventional lithium-ion batteries, the direct reaction between oxygen and light metals such as lithium and sodium in metal–oxygen systems circumvents the need for a heavy transition metal redox couple in their operation, thereby making a high gravimetric energy density achievable [3] , [4] , [5] , [6] , [7] . The most intensively studied metal–oxygen system to date is the lithium–oxygen (Li–O 2 ) battery, which shares a similar lithium chemistry with lithium-ion batteries. However, this system suffers from poor cycle stability and efficiency, which has retarded the feasibility of its use in practical systems [8] , [9] . In particular, the large charge overpotential over 1 V, the main reason for the low efficiency, also accelerates the degradation of the electrode and electrolyte [9] . As an alternative, Na has been introduced to replace Li in Li–O 2 batteries with a few important merits [10] . Despite the reduction in the energy density resulting from the lower redox potential of Na/Na + , Na resources are readily available, are less expensive than Li and can easily replace Li in the battery chemistry. It has been reported that the redox reactions in the sodium–oxygen (Na–O 2 ) battery result in an extremely low charge overpotential ( ∼ 0.2 V) despite involving the formation of micrometre-sized sodium superoxide (NaO 2 ) cubic crystallites [11] , [12] , [13] , [14] . This unique phenomenon supports the idea that this system is a promising alternative not only in terms of the cost of materials but also regarding the potential practical performance advantages. Notably, however, the reactions of Na–O 2 cells appear to be more diverse than those of Li–O 2 cells. Contrary to the initial report of NaO 2 discharge products, some recent lines of work could not reproduce either the formation of the discharge product NaO 2 or the low charge overpotential [15] , [16] , [17] . It was reported that sodium peroxide (Na 2 O 2 ) [15] , [16] , [17] or sodium peroxide dihydrate (Na 2 O 2 ·2H 2 O) [18] , [19] was formed instead. In addition, these cells exhibited high overpotential during charge, similar to that observed in the Li–O 2 system. Many groups have attempted to determine the reasons for these discrepancies; however, to date, the main cause of the divergence of reactions has not been identified. Janek et al . investigated the effect of different carbon electrodes; Guo et al . and Shao-Horn et al . addressed this issue but observed no critical differences among the cases [12] , [20] , [21] . In this work, we demonstrate the interplay of the diverse reactions in Na–O 2 batteries involving a series of electrochemical and chemical reactions as a function of time. Under systematic control of the operating conditions, we observe that the galvanostatic charge/discharge profiles are sensitively affected by the conditions and durations of the electrochemical operations. It is also revealed that the electrochemically formed NaO 2 is unstable and degrades into Na 2 O 2 ·2H 2 O in the absence of an applied current. The spontaneous dissolution and ionization of NaO 2 liberates the free O 2 − in the electrolyte and promotes side reactions involving the formation of Na 2 O 2 ·2H 2 O. On the basis of these observations, we propose reaction mechanisms of Na–O 2 batteries under various operating conditions. This report is the first to reveal the relationships among the different discharge products observed in Na–O 2 batteries, which broadens our understanding of the electrochemical and chemical reactions in Na–O 2 batteries. Furthermore, these discussions may offer insight and guidance to the metal–air battery community in terms of regulating the kinetics of the intertwined reactions. Electrochemical profile depending on the operating condition To address the previous conflicting results on the discharge products and overpotentials of Na–O 2 cells, we carefully assessed the effects of operating parameters on the resulting electrochemical profiles. Among the various parameters examined ( Supplementary Figs 1–3 and Supplementary Notes 1–3 ), we observed that the charge/discharge profiles were most sensitively affected by the applied current and rest time between the discharge and charge, which was analogous to the report by Yadegari et al . as a function of discharge current or limited capacities [19] . 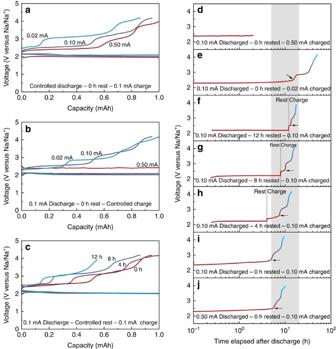Figure 1: Electrochemical charge/discharge profiles of Na–O2cells under various operating conditions. (a) Discharge currents of 0.02, 0.1 and 0.5 mA; (b) charge currents of 0.02, 0.1 and 0.5 mA and (c) rest times of 0, 4, 8 and 12 h. All the cells utilized a limited capacity of 1.0 mAh. (d–j) Representations of voltage profiles as a function of time corresponding toa–c. The shaded area indicates that range of the first points of the polarized charge potentials. Figure 1 presents and compares the electrochemical profiles obtained under various conditions. Although the discharge profiles are similar, with a single plateau at ∼ 2.1 V, there are roughly three different charging plateaus observed at (i) ∼ 2.5 V, (ii) ∼ 3.0 V and (iii) 3.8 V, which agree with recent reports under certain settings [19] , [20] . However, the relative lengths of each plateau markedly vary under differing operating conditions. For the cases of controlled discharge currents followed by a constant current charging in Fig. 1a , it was observed that the length of the lower plateau ( ∼ 2.5 V) in the charge profiles was reduced as the applied discharge current decreased from 0.5 to 0.02 mA. However, the lengths of the plateaus at higher voltages, that is, ∼ 3.0 and 3.8 V, were substantially increased, resulting in an overall larger overpotential. Similar behaviours were observed in Fig. 1b when varying the charge currents after a constant current discharge. With the lower applied charge currents, the cell exhibited a higher charging overpotential with shortened plateau length at 2.5 V. This result contrasts with the general observation that slow charging/discharging of electrochemical cells results in a voltage close to the equilibrium potential, thereby resulting in smaller overpotentials. In addition, this result strongly indicates that the different discharge products might undergo the charging process at each case. Notably, the shapes of the electrochemical charge profiles provide important clues to determine the discharge products of Na–O 2 reactions [19] , [22] . Even though the discharge products should be identical for the cases of the same protocol of discharge, each charge profile was distinct with different charge currents. This finding implies that the initial discharge products are gradually transformed into other phases during the charge process via time-dependent reactions. To verify whether this transformation occurs via an electrochemical or chemical reaction, we also controlled the rest time between the discharge and charge processes. As observed in Fig. 1c , the lowest voltage region in the charge profiles systematically decreases on increasing the rest time from 0 to 12 h. The change in the electrochemical profile in the absence of the applied current clearly indicates that the time-dependent chemical reactions occurred during the rest period, affecting the subsequent charging. This behaviour was also confirmed in similar tests for the higher charging currents with the resting time after the discharge, which revealed the growth of the charge polarizations on increasing the rest time ( Supplementary Fig. 1 ). Figure 1: Electrochemical charge/discharge profiles of Na–O 2 cells under various operating conditions. ( a ) Discharge currents of 0.02, 0.1 and 0.5 mA; ( b ) charge currents of 0.02, 0.1 and 0.5 mA and ( c ) rest times of 0, 4, 8 and 12 h. All the cells utilized a limited capacity of 1.0 mAh. ( d – j ) Representations of voltage profiles as a function of time corresponding to a – c . The shaded area indicates that range of the first points of the polarized charge potentials. Full size image The time-dependent chemical reactions can be more clearly visualized by plotting all the voltage profiles as a function of the time. Figure 1d–j illustrates the voltage evolution of each cell after the completion of the discharge at different operating conditions. The first inflection points of the voltage profiles at charge (indicated with arrows) occur at ∼ 10 h regardless of the rest or charge protocols. This result indicates that a specific time of ∼ 10 h is required before observing a change of the profile, which hints at the kinetics of the chemical reactions. Time-resolved characterization of discharge products To confirm the time-dependent phase transformation of the discharge products via chemical reaction in Na–O 2 cells, we characterized the discharge products in air electrodes as a function of the rest time. The highly crystalline NaO 2 was observed directly after the discharge with no other phases, as demonstrated in the X-ray diffraction spectra ( Fig. 2a,b ) [11] . However, after being aged for several hours, the NaO 2 peak slowly diminished, whereas the characteristic peak of Na 2 O 2 ·2H 2 O began to appear and grew. After 12 h of resting, the initial discharge product was completely transformed into Na 2 O 2 ·2H 2 O. It should be noted that Na 2 O 2 ·2H 2 O has often been regarded as a main discharge product in previous reports of Na–O 2 batteries [18] , [19] , [20] . Recently, Ortiz-Vitoriano et al . reported that NaO 2 could convert to Na 2 O 2 ·2H 2 O on exposure to the ambient air during the characterization at room temperature [21] . However, our data show that such transformation occurs in the electrochemical cells by the intrinsic dissolving characteristics of NaO 2 in the electrolyte even without the exposure to the ambient atmosphere. Remarkably, the time taken for the discharge product to completely transform into Na 2 O 2 ·2H 2 O coincides with the timeline of Fig. 1d–j , which shows the inflection of the voltage rising after ∼ 10 h. When we analysed the phases of the discharge products as a function of the applied discharge currents ( Supplementary Fig. 4 ), it was also observed that the NaO 2 /Na 2 O 2 ·2H 2 O ratio decreased with the lower operating current, which is consistent with the time-dependent transformation of the discharge products. 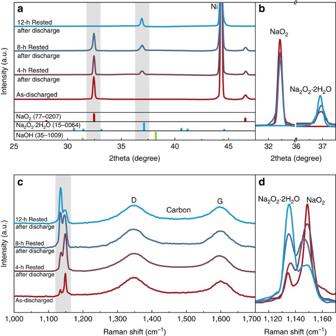Figure 2: Time-resolved characterization showing the phase transitions of the discharge products of the Na–O2cells. (a,b) X-ray diffraction spectra of the discharged cathodes of Na–O2batteries with rest times of 0, 4, 8 and 12 h. (c,d) Raman spectra of the discharged cathodes of Na–O2batteries with rest times of 0, 4, 8 and 12 h. Figure 2: Time-resolved characterization showing the phase transitions of the discharge products of the Na–O 2 cells. ( a , b ) X-ray diffraction spectra of the discharged cathodes of Na–O 2 batteries with rest times of 0, 4, 8 and 12 h. ( c , d ) Raman spectra of the discharged cathodes of Na–O 2 batteries with rest times of 0, 4, 8 and 12 h. Full size image Raman spectroscopy results confirmed that the initial NaO 2 discharge products gradually transformed into Na 2 O 2 ·2H 2 O with resting. In Fig. 2c , the two distinct peaks of NaO 2 and Na 2 O 2 ·2H 2 O are detected along with the characteristic bands (D/G) of the carbon electrode. The Raman signals at 1,156 and 1,136 cm −1 are attributed to the O–O stretch bonding in NaO 2 and Na 2 O 2 ·2H 2 O, respectively [21] . The systematic change in the relative ratios of NaO 2 and Na 2 O 2 ·2H 2 O with time is clearly illustrated in Fig. 2d , which agrees well with the results in Fig. 2b . The phase transition of NaO 2 to proton-containing Na 2 O 2 ·2H 2 O indicates a source of protons in the electrochemical cell. Considering the low water content in the electrolyte used for the cell (less than ∼ 5 p.p.m. ), which is insufficient to form the phase (calculations provided in Supplementary Note 4 ) [21] , [23] , [24] , the protons are likely delivered from other sources such as the electrolyte solvent. As we could expect, the rechargeability of Na–O 2 cell was better for the highly biased electrochemical conditions coupled with the low polarized charge profile ( Supplementary Fig. 3 ), which is attributed to the electrochemical formation and decomposition of NaO 2 as shown in Supplementary Fig. 5 . However, the electrochemical reversibility with the three-stepped charge profile shown from Na 2 O 2 ·2H 2 O was relatively worse compared with the former conditions. The proposed transformation mechanism will be discussed in detail later. Morphological change of discharge products over time To visualize the transition process, we examined the morphologies of the discharge products at different rest times within 12 h. In Fig. 3a , well-defined micron-sized cubic NaO 2 was observed immediately after the discharge, which agrees with the observation of Hartmann et al . [11] . However, the edges of the cubes became significantly dull, and the overall shapes of the cubes obtained were smudged during the rest period ( Fig. 3b,c ). At the end of the rest period, the cubic crystallites completely disappeared, and rod-shaped microparticles began to appear, which resemble the Na 2 O 2 ·2H 2 O in a previous report [19] . This morphological change suggests the disappearance of NaO 2 and the subsequent appearance of Na 2 O 2 ·2H 2 O in the cell during the rest period. Moreover, this finding implies that the transformation does not occur via a conventional solid-state or interfacial reaction between NaO 2 and the electrolyte to form Na 2 O 2 ·2H 2 O, which would not involve significant morphological change. Rather, it is likely to be a solution-mediated process through dissolution and nucleation [25] , [26] , [27] . 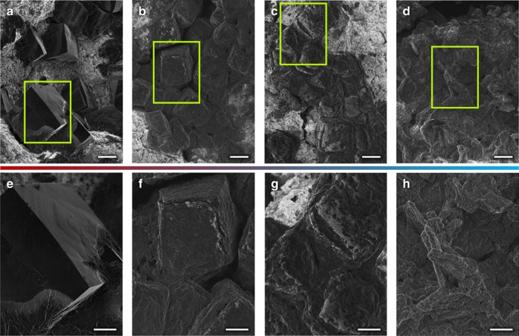Figure 3: Time-resolved examinations of the morphology of discharge products on the cathodes of Na–O2cells. (a–d) Morphology of the discharge products of Na–O2cells (scale bar, 10 μm). (e–h) Corresponding magnified scanning electron microscopy micrographs (scale bar, 5 μm); (a,e) as-discharged, (b,f) 4-h rest after discharge, (c,g) 8-h rest after discharge and (d,h) 12-h rest after discharge. Figure 3: Time-resolved examinations of the morphology of discharge products on the cathodes of Na–O 2 cells. ( a – d ) Morphology of the discharge products of Na–O 2 cells (scale bar, 10 μm). ( e – h ) Corresponding magnified scanning electron microscopy micrographs (scale bar, 5 μm); ( a , e ) as-discharged, ( b , f ) 4-h rest after discharge, ( c , g ) 8-h rest after discharge and ( d , h ) 12-h rest after discharge. Full size image Dissolution and ionization of NaO 2 We investigated the possibility of the dissolution of the solid NaO 2 phase in the electrolyte using electron spin resonance (ESR) spectroscopy, which is useful for detecting the magnetic responses of the unpaired electrons in radicals such as O 2 − (ref. 28 ). Surprisingly, as observed in Fig. 4a , with the simple immersion of the pre-discharged cathodes, the ESR signal evolved within 10 min from the fresh electrolyte, indicating the presence of O 2 − . To avoid any effect of the remaining oxygen from the disassembled Na–O 2 cells, the pre-discharged cathodes were washed with fresh electrolyte before the measurement, which led to an identical result. The calculated g -value of 2.0023 for the observed ESR signal corresponds well with the theoretical value of the unpaired electron in free O 2 − (ref. 29 ). The solubility of NaO 2 in the electrolyte was roughly estimated to be ∼ 187 mM, which is in the similar order with the report by Schechter et al . [30] , but has a relatively large discrepancy to the report by Hartmann et al . [31] . This discrepancy might be mainly due to the additional chemical reactions involving the precipitation of solid Na 2 O 2 ·2H 2 O. The detection of O 2 − indicates that the NaO 2 is soluble in the ether-based electrolytes, which was also expected from the literatures with the electrochemical determinations [21] , [24] , [31] . Furthermore, this behaviour is analogous to highly soluble LiO 2 in the solvatable conditions of Li–O 2 batteries [23] , [32] . More importantly, the dissolution can immediately lead to the ionization of NaO 2 , liberating O 2 − , the consequences of which will be discussed later. 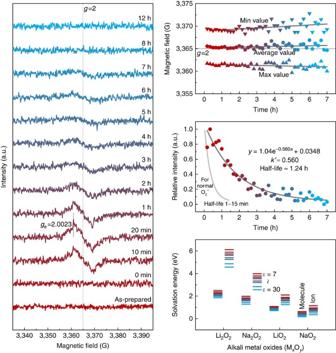Figure 4: ESR analysis and theoretical calculations of the dissolution and ionization of NaO2into the electrolyte. (a) Time-dependent ESR measurements for the fresh electrolytes (0.5 M NaCF3SO3in diethylene glycol dimethyl ether) with soaking of the pre-discharged cathode without any aging. (b) Maximum, minimum and average values of ESR signals as a function of time. (c) Exponential decay of ESR signals and the common trend line of O2−. (d) Calculations of the solvation energy for several alkali-metal superoxides and peroxides with the various dielectric constants (ɛ=7∼30). Figure 4: ESR analysis and theoretical calculations of the dissolution and ionization of NaO 2 into the electrolyte. ( a ) Time-dependent ESR measurements for the fresh electrolytes (0.5 M NaCF 3 SO 3 in diethylene glycol dimethyl ether) with soaking of the pre-discharged cathode without any aging. ( b ) Maximum, minimum and average values of ESR signals as a function of time. ( c ) Exponential decay of ESR signals and the common trend line of O 2 − . ( d ) Calculations of the solvation energy for several alkali-metal superoxides and peroxides with the various dielectric constants ( ɛ =7 ∼ 30). Full size image Figure 4b shows that the peak widths of the ESR signals increased slightly with time. The broadening indicates the energy exchange of the spin with the local environments via spin–spin relaxation or spin–lattice relaxation [28] . This interaction supports the time-dependent chemical reactions associated with the dissolved O 2 − with its neighbouring electrolyte solvent. The intensity of the O 2 − signal is the highest ∼ 20 min after the immersion and exponentially decreases over time, indicating the instability of O 2 − in the electrolyte [33] . From this behaviour, we could derive that it was a pseudo-first-order reaction that mainly relates with the concentration of O 2 − . On the basis of the exponential fitting of the relative intensity of ESR signals, the pseudo-first-order rate constant of H + abstraction was obtained as ∼ k ′≈0.560, and its corresponding half-life was estimated as ∼ t 1/2 =ln (2)/ k ′≈1.24 h (the detailed derivation is in Supplementary Note 5 ). Figure 4c reveals, however, that the time-dependent decay of the intensity is relatively sluggish compared with the intrinsic lifetime of normal O 2 − . Typically, the half-life of O 2 − is ∼ 1–15 min because of its high reactivity and instability [34] . The abnormally long half-life in the electrolyte ( ∼ 1.24 h) in our case is believed to occur because O 2 − is continuously generated with the dissolution of NaO 2 . The ESR signal completely vanished after ∼ 8 h, which is slightly faster than the time required for the formation of Na 2 O 2 ·2H 2 O in Fig. 2 . Despite the evolution of O 2 − , the overall signal decay might be induced from the relatively dominant H + abstraction due to the reactivity of O 2 − . This gap in the kinetics might originate from the time required to form the Na 2 O 2 ·2H 2 O phase from the O 2 − . To understand the dissolution and ionization behaviour of NaO 2 , the solvation energies of various alkali-metal superoxides and peroxides were calculated for comparison using first-principle calculations with the series of dielectric constant from 7 to 30. Figure 4d reveals that generally the superoxide exhibits a lower solvation energy than the peroxide for both lithium and sodium compounds. This result is consistent with our result of NaO 2 dissolution and the recent experimental findings for Li–O 2 batteries, which indicated that LiO 2 is found mostly as soluble intermediates in the electrolyte in contrast to the solid phase of Li 2 O 2 (refs 23 , 32 ). In addition, it is notable that the solvation energy of the sodium phases was significantly lower than that of the lithium phases, which is attributed to the weaker Lewis acidity of the Na cation compared with that of the Li cation in the polar solvent [35] , [36] . However, for the solvents with substantially lower dielectric constant ( ɛ = ∼ 7), the dissolution is not favourable even in NaO 2 . Molecular dissolution energies of NaO 2 in model solvents are ∼ 0.6 eV, which roughly corresponds to one molecule dissolution among 10 10 formula units of NaO 2 . On the other hand, it markedly diminishes to 0.17 eV (one molecule among 10 3 formula units of NaO 2 ) in ɛ =30 (ref. 37 ). Note that, for the low dielectric constant solvents, dielectric constant of the solution sensitively increases with increasing salt concentration, which can result in higher solution dielectric constant than that of the pure solvent [38] . Therefore, it is expected that the dissolution of NaO 2 can occur when salts are present in the electrolyte, which is consistent with the observation of O 2 − in the ESR analysis. It also is noted that even with the dissolving characteristics of NaO 2 , the crystallization of NaO 2 is possible in the normal discharging conditions with the supersaturation of localized reactants such as Na + and O 2 − (refs 21 , 31 , 39 , 40 ). In the other case where the supply of the reactants such as Na + is limited, for example, in the absence of the applied voltage, the dissolution and ionization might dominate, giving rise to the formation of Na 2 O 2 ·2H 2 O as a discharge product. Proposed mechanism of Na–O 2 batteries On the basis of the previous reports and our new findings, we propose a mechanism that describes the electrochemical and chemical reactions in Na–O 2 systems in Fig. 5 . The well-established discharge process [11] can be illustrated with the reduction of an O 2 molecule into O 2 − , which reacts with Na + to form NaO 2 (Reaction 1), and the charge process is the reverse reaction (Reaction 2). After or during the discharge, the NaO 2 is prone to dissolution and ionization into the electrolyte based on the solvating energy ( ΔG sol ) in the solvent (Reaction 3) [32] . The dissolution of NaO 2 generates O 2 − , which can degrade the surrounding molecules because of its chemical instability. Typically, the liberated O 2 − is a strong reagent for the abstraction of H + from the electrolyte solvents (Reaction 4) [9] , and the degree of H + abstraction [41] , [42] is determined by the acid-dissociation constant (p K a ) of the solvent. Some hydroperoxyl radicals (HO 2 ) might be formed during this process, resulting in the nucleophilic attack of the H + -lost solvent (Reaction 5) [43] . However, the evolution of HO 2 can be helpful in promoting the solution-mediated discharge/charge process as recently reported by Xia et al . [24] . Nevertheless, in a circumstance where the dissolution/ionization of NaO 2 is dominant, the liberation of O 2 − is overwhelmingly larger than a possible HO 2 formation, inducing the H + abstraction from the neighbouring electrolyte solvent. Meanwhile, the solvent undergoes oxidative decompositions to produce byproducts such as carbon dioxide (CO 2 ), water (H 2 O) and hydroxyl anions (OH − ; Reaction 6) [9] . It is also possible that the coupling of HO 2 leads to disproportionation into hydrogen peroxide (H 2 O 2 ) and O 2 (Reaction 7) [44] . In the presence of both Na + and OH − , which is effectively the dissolution state of sodium hydroxide (NaOH), a solid crystallite of NaOH can precipitate with a higher concentration of OH − produced. Further reaction between NaOH and H 2 O 2 from Reaction 7 leads to the formation of Na 2 O 2 ·2H 2 O via peroxo-hydroxylation, whose reverse reaction is well known (Reaction 8) [45] . To support our proposed reaction mechanism, we chose several intermediate reactions that should be verified according to the reaction model in the Supplementary Information . Supplementary Figs 6–9 demonstrate that O 2 − plays an important role after the dissolution of NaO 2 in converting the discharge product to Na 2 O 2 ·2H 2 O via degradation of the electrolyte involving OH − and H 2 O 2 . These identifications strongly support the proposed mechanism of competing electrochemical and following chemical reactions in Na–O 2 batteries. The detailed discussions are provided in Supplementary Notes 6–9 . 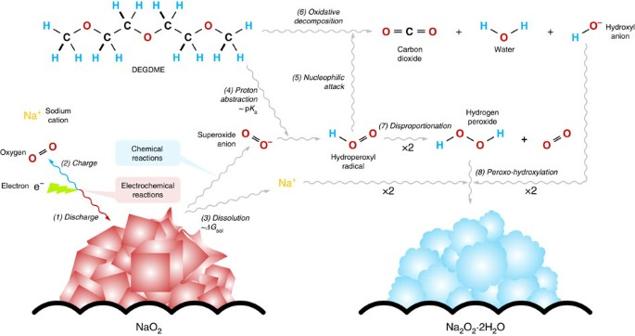Figure 5: Schematic of the proposed mechanism illustrating the electrochemical and chemical reactions under various operating conditions. For the electrochemical reaction, NaO2is formed and decomposed during discharge/charge (Reactions 1 and 2). For the chemical reaction, NaO2is dissolved and ionized into the electrolyte (Reaction 3), which promotes the undesired degradation of the electrolyte (Reactions 4–6). Na2O2·2H2O is formed during the subsequent chemical reactions (Reactions 7 and 8). The reaction equations are summarized below: Figure 5: Schematic of the proposed mechanism illustrating the electrochemical and chemical reactions under various operating conditions. For the electrochemical reaction, NaO 2 is formed and decomposed during discharge/charge (Reactions 1 and 2). For the chemical reaction, NaO 2 is dissolved and ionized into the electrolyte (Reaction 3), which promotes the undesired degradation of the electrolyte (Reactions 4–6). Na 2 O 2 ·2H 2 O is formed during the subsequent chemical reactions (Reactions 7 and 8). Full size image It is noteworthy that a similar behaviour has been recently reported for reactions in Li–O 2 batteries. The solvating environment was demonstrated to alter the stability of the intermediates, such as a lithium superoxide (LiO 2 ), thus affecting the overall reaction paths [23] , [32] . LiO 2 is a precedent phase with the direct reaction of a Li cation and superoxide anion (O 2 − ), which readily decomposes into lithium peroxide (Li 2 O 2 ) via either an electrochemical surface reaction or disproportionation [23] , [32] . Although LiO 2 is known to be unstable [46] , [47] , it was recently demonstrated that LiO 2 might be dissolved into the electrolyte and aid in the formation of the toroidal Li 2 O 2 via a solution reaction under highly solvating conditions [23] . NaO 2 shares this dissolving nature with LiO 2 even though the thermodynamic stability of NaO 2 warrants its formation as a discharge product. The significant dissolution of NaO 2 supports the conclusion that the dominant reaction in Na–O 2 batteries relies on the solution-mediated reactions of nucleation and growth of NaO 2 (refs 21 , 24 , 31 ) and implies that the capacities and morphology of the reaction products would be greatly affected by the energetics of NaO 2 under various conditions (such as different electrolytes and current rates). This is also supplemented with the recently reported observations [21] , [31] and operating mechanism [24] in terms of the various states of electrochemical and chemical reactions. We successfully demonstrated the interplay of the diverse competing reactions in Na–O 2 batteries. The time-dependent chemical reactions were identified as being triggered from the dissolution and ionization of the electrochemically formed NaO 2 in the electrolyte. The liberated O 2 − reacts with the electrolyte solvent to form Na 2 O 2 ·2H 2 O following a series of intermediate steps. The Na 2 O 2 ·2H 2 O in the air electrode requires a higher energy for the decomposition, which leads to the increased charge overpotential and irreversibility of Na–O 2 cells. This report is the first to correlate the electrochemical and chemical reactions with the operating conditions in Na–O 2 batteries, and our findings concerning the relationships among different phases resolve the conflicting observations of different discharge products in previous Na–O 2 batteries. To prepare a better performing Na–O 2 battery, a strategy to prevent the transformation of NaO 2 into Na 2 O 2 ·2H 2 O while still allowing the solution-mediate discharge reaction is necessary. We hope that the findings of this study can provide a basis for researchers to navigate and direct the reactions in Na–O 2 batteries to achieve high efficiency and rechargeability. Cell assembly and galvanostatic cycling of Na–O 2 cells The carbon cathode was prepared by casting Ketjen Black carbon paste and polytetrafluoroethylene (60 wt% emersion in water, Sigma-Aldrich) with a mass ratio of 9:1 in a solution of isopropanol (>99.7%, Sigma-Aldrich) and N-methyl-2-pyrrolidone (99.5%, anhydrous, Sigma-Aldrich) with a volume ratio of 1:1 on Ni mesh current collectors. The carbon-coated Ni mesh was dried at 120 °C and heated at 400 °C for 4 h in Ar to completely remove any residual H 2 O impurities. All the procedures described below were performed in an Ar-filled glove box (O 2 level<0.5 p.p.m. and H 2 O level<0.5 p.p.m.). The Na–O 2 cells were assembled as a Swagelok-type cell with stacking of the Na metal anode, electrolyte-soaked separators and carbon cathode, which was punched with a half-inch diameter. The Na metal anode was carefully prepared by milling dry Na metal chunks (ACS Reagent, Sigma-Aldrich) after removing the contaminated surfaces. The electrolyte was prepared with diethylene glycol dimethyl ether (anhydrous, 99.5%, Sigma-Aldrich), which contains 0.5 M NaCF 3 SO 3 (98%, Sigma-Aldrich). The solvent was dried using 3-Å molecular sieves for over 1 week, and the salt was also kept in a vacuum oven at 180 °C for the same time before use. The final water content in the electrolyte was less than 10 p.p.m. according to a Karl–Fisher titration measurement. The amount of electrolyte used for the cell was 200 μl. Two sheets of Celgard 2400 were used as separators. Electrochemical battery tests of the Na–O 2 cells were conducted using a potentio-galvanostat (WonA Tech, WBCS 3000, Korea). All the cells were relaxed under 770 torr of O 2 pressure for 10 min before the tests. After being saturated with O 2 gas, the cells were operated in the closed state with a limited capacity of 1 mAh, lower voltage cutoff of 1.6 V and upper voltage cutoff of 4.2 V. Special protocol based on a pulsed current was applied during the charge to avoid dendritic failure of the Na metal anode. The on/off time ratio of the pulse charge was 1:4 (applying current for 0.5 s and relaxing for 2 s). More details about our charge protocol are provided in Supplementary Figs 10 and 11 and following discussions in Supplementary Note 10 . Characterization of Na–O 2 cells The discharged cathodes after the different rest times were collected from disassembled Na–O 2 cells and washed with acetonitrile (anhydrous, 99.8%, Sigma-Aldrich) in a glove box to remove any residual electrolyte. X-ray diffraction spectra of the cathodes were obtained using a Bruker D2-Phaser (Cu Kα λ =1.5406 Å) with the aid of a specially designed air-tight holder to prevent outer atmospheric contamination. Raman spectra were obtained using a Horiba Jobin-Yvon LabRam Aramis spectrometer (the 514-nm line of an Ar–ion laser was used as the excitation source). The scattered light of the Raman signal was collected in a backscattering geometry using the × 50 microscope objective lens. Field-emission scanning electron microscopy (MERLIN Compact, ZEISS, Germany) was used for the morphological observations after Pt coating. For ESR characterization, the collected powder from the discharged cathodes after rinsing to remove the residual used electrolytes was soaked in fresh electrolyte. After immersing the powdery discharged cathodes, the ESR signal of the electrolytes was measured at room temperature using a JEOL JES-TE200 ESR spectrometer every 10 min for 12 h using a liquid quartz cell. The microwave X-band frequency was 9.42 GHz at 1-mW power. Theoretical calculations of solvation energy First-principles calculations were performed using the spin-polarized generalized gradient approximation. A continuum solvation model (VASPsol [48] , [49] code) was used to evaluate the solvation energy of the alkali-metal superoxide/peroxide (M x O 2 , M: Li, Na, x =1 or 2). The following equations were used considering both the (1) molecular and (2) ionized solvated states: where E solvated (M x O 2 ) and E bulk (M x O 2 ) are the total energies of the solvated and bulk M x O 2 per formula unit, respectively. The solvated species (ions or molecules) were placed in a 13 Å × 13 Å × 13 Å cell as an isolated species. We used the plane-wave basis with an energy cutoff of 550 eV and a Monkhorst-Pack 2 × 2 × 2 k -point mesh. On the basis of previous reports [50] , [51] that stated that the solvation entropy term (TS) of polar molecules and ions in the standard state is less than 5% of the enthalpy term ( H ), we neglected the entropy effect of the solvation in these calculations. How to cite this article: Kim, J. et al . Dissolution and ionization of sodium superoxide in sodium–oxygen batteries. Nat. Commun. 7:10670 doi: 10.1038/ncomms10670 (2016).